Constitutively active Foxo3 in oocytes preserves ovarian reserve in mice During female reproductive life, ovarian follicle reserve is reduced by maturation and atresia until menopause ensues. Foxo3 is required to maintain the ovarian reserve in mice. Here we show that overexpression of constitutively active FOXO3 can increase ovarian reproductive capacity in mice. We find increased follicle numbers and decreased gonadotropin levels in aging FOXO3 -transgenic mice compared with wild-type littermates, suggesting maintenance of a greater ovarian reserve. Based on cumulative progeny in aging animals, we find 31–49% increased fertility in transgenic females. The gene expression profile of Foxo3−/− knockout ovaries appears older than that of wild-type littermates, and the transgene induces a younger-looking profile, restoring much of the wild-type transcriptome. This is the first gain-of-function model of augmented reproductive reserve in mice, thus emphasizing the role of Foxo3 as a guardian of the ovarian follicle pool in mammals and a potential determinant of the onset of menopause. Resting (non-growing) primordial follicles comprise the ‘ovarian reserve’, the size of which is a critical indicator of female fertility and the approximate determinant of reproductive lifespan [1] . In women, the number of primordial follicles decreases from about 700,000 at the end of folliculogenesis [2] to about 1,000 when menopause ensues about age 51 (ref. 3 ). The initial pool of primordial follicles progressively decreases as follicles are recruited for ovulation [1] . These processes are strictly regulated to prevent premature exhaustion of the primordial follicle reservoir (premature ovarian failure) [4] . Premature ovarian failure, defined by menopause before age 40, affects about 1% of women [5] . How follicle recruitment is regulated is still largely unknown, but the forkhead transcription factor FOXO3 is strongly implicated. When Foxo3 was ablated in mice, primordial follicles underwent massive and uncontrolled activation, leaving the ovary virtually empty and the females sterile by the age of 15 weeks [6] . This showed that Foxo3 is required to maintain the follicle reserve pool. FOXO3 activity is regulated by phosphorylation: the unphosphorylated form is transcriptionally active in the nucleus; upon phosphorylation, the protein is exported to the cytoplasm, thereby losing transcriptional activity [7] . In the mouse ovary, cytoplasmic export of Foxo3 in the oocytes coincides with the recruitment of follicles [7] . Here, we test if this regulatory step is critical for follicle recruitment, that is, if FOXO3 function in the nucleus helps to maintain the follicle reserve pool. We generate a mouse model harbouring a FOXO3 gene that lacks critical phosphorylation sites and is thus constitutively active in the nucleus. These sites have been described as involved in the inactivation of Foxo3 through phosphorylation by kinases such as Akt, Sgk, Ck1 and Dyrk1 [8] , [9] . FOXO3 -transgenic female mice show less increase in gonadotropin levels than age-matched wild-type animals, and display enhanced fertility. Consistent with these findings, the number of ovarian follicles is larger in FOXO3 -transgenic mice throughout their fertile life. Finally, gene expression analyses suggest the maintenance of a younger profile in the presence of the transgene. These results support a role of Foxo3 in maintaining the ovarian reserve, and thereby regulating the reproductive capacity of the female mouse. Expression of transgenic FOXO3 This FOXO3 transgene was placed under the control of a Kit promoter, assuring high expression in oocytes at the primordial and primary follicle stage [10] ( Fig. 1a ). We verified the expression of the transgenic FOXO3 specifically by real-time PCR with construct-specific primers at birth (P0), 7 and 21 days (P7 and P21) ( Fig. 1b ). As follicle formation and maturation progressed, the level of FOXO3 decreased over time ( Fig. 1b ). However, Foxo3 levels remained consistently higher in the transgenic ovaries when assayed with primers that detected both endogenous and transgene messenger RNA ( Fig. 1c ). The ratio of the expression of Foxo3 in transgenic/wild-type ovaries remained constant at 1.44±0.08. Protein expression was also evaluated by western blot ( Fig. 1d ) at P7 and P21. Expression of FOXO3 was again confirmed with a stronger signal in the transgenic ovaries by band intensity analysis, thus consistent with RNA results (ratio of FOXO3 protein in transgenic/wild-type ovaries was 1.48 at P7 and 3.59 at P21). 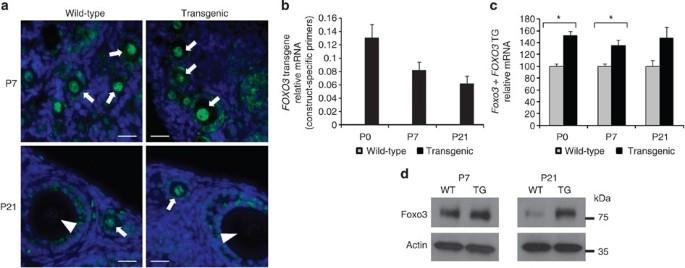Figure 1: Foxo3 expression in wild-type and transgenic ovaries. (a) Immunostaining for FOXO3 in wild-type andFOXO3-transgenic ovaries at age 7 and 21 days. For both genotypes, the signal is strong in oocyte nuclei from primordial and primary follicles (arrows) and is lost upon differentiation into secondary follicles (arrowheads). Nuclei are stained blue with DAPI. Bar, 20 μm. (b) Expression ofFOXO3transgene by real-time PCR using construct-specific primers in wild-type (grey, no signal as expected) and transgenic (black) ovaries (n=3 per genotype) at P0, P7 and P21. (c) Expression of totalFoxo3by real-time PCR using primers that amplified both the transgene and the endogenousFoxo3,showing increased cumulative expression in transgenic ovaries (n=3 per genotype). (d) Western blot confirming an increased expression of FOXO3 in P7 and P21 transgenic ovaries compared with wild-type. Actin was used as loading control. Data in panels (b–c) are represented as mean values±s.e.m. *P<0.05, unpairedt-test. P0, 0 dpn; P7, 7 dpn; and P21, 21 dpn. Figure 1: Foxo3 expression in wild-type and transgenic ovaries. ( a ) Immunostaining for FOXO3 in wild-type and FOXO3 -transgenic ovaries at age 7 and 21 days. For both genotypes, the signal is strong in oocyte nuclei from primordial and primary follicles (arrows) and is lost upon differentiation into secondary follicles (arrowheads). Nuclei are stained blue with DAPI. Bar, 20 μm. ( b ) Expression of FOXO3 transgene by real-time PCR using construct-specific primers in wild-type (grey, no signal as expected) and transgenic (black) ovaries ( n =3 per genotype) at P0, P7 and P21. ( c ) Expression of total Foxo3 by real-time PCR using primers that amplified both the transgene and the endogenous Foxo3, showing increased cumulative expression in transgenic ovaries ( n =3 per genotype). ( d ) Western blot confirming an increased expression of FOXO3 in P7 and P21 transgenic ovaries compared with wild-type. Actin was used as loading control. Data in panels ( b – c ) are represented as mean values±s.e.m. * P <0.05, unpaired t -test. P0, 0 dpn; P7, 7 dpn; and P21, 21 dpn. Full size image Ovarian reserve retention is increased in FOXO3 mice We next assessed the effects of the transgenic FOXO3 on follicle dynamics and ovarian aging. As menopause is preceded by a rise in follicle-stimulating hormone (FSH) and luteinizing hormone (LH) [11] , we investigated whether follicle depletion occurred more slowly in transgenic female mice. Serum concentrations of gonadatropins FSH and LH were, as expected, increased in 9-month-old female mice compared with younger mice ( Fig. 2a ), but were significantly lower in 9-month-old transgenic animals compared with age-matched wild-type (stratified t -test, P -value <0.001 for both parameters). In addition, in contrast to their 9-month wild-type counterparts, LH levels of 9-month transgenic females were nearly identical to the younger, 3-month wild-type females ( Fig. 2b ). 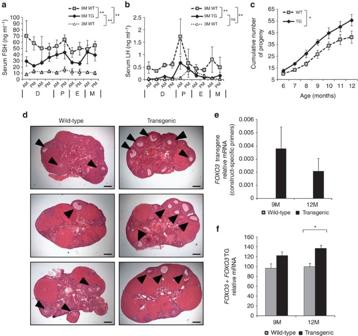Figure 2: Fertility measures and morphology ofFOXO3-transgenic ovaries. (a) Serum FSH and (b) serum LH in 9-month-old wild-type and transgenic mice (n=3 per genotype). The level in young (3-month-old) wild-type mice is also shown as a reference (n=3). (c) Cumulative number of pups are greater in transgenic animals compared with wild-type through 12 months of age (n=4 per genotype). (d) Appearance of aged wild-type and transgenic ovaries (12 months). The middle section of each ovary was photographed for an unbiased comparison. Transgenic ovaries retain a larger pool of follicles appearing more active in folliculogenesis with antral follicles (arrowheads) that are more abundant in the transgenic ovaries, whereas wild-type ovaries are filled with corpora lutea. (e) Expression of theFOXO3transgene by real-time PCR using construct-specific primers in wild-type (grey, no signal as expected) and transgenic (black) ovaries (n=4 per genotype) at 9 and 12 months of age. (f) Expression of totalFoxo3by real-time PCR using primers common for both the transgene and the endogenousFoxo3,showing increased cumulative expression in transgenic ovaries (n=4 per genotype). Data of panels (a–c;e–f) are represented as mean values±s.e.m. *P<0.05; **P<0.001; NS=not significant (P>0.05). A stratifiedt-test was used for panelsaandb; a linear mixed-effect model was used for panelc; and unpairedt-test was used for panelseandf. AM, morning; D, dioestrus; E, oestrus; M, metestrus; P, proestrus; PM, evening; TG, transgenic; WT, wild-type; 3M, 3 months; 9M, 9 months; 12M, 12 months. For paneld, bar, 0.2 mm. Figure 2: Fertility measures and morphology of FOXO3 -transgenic ovaries. ( a ) Serum FSH and ( b ) serum LH in 9-month-old wild-type and transgenic mice ( n =3 per genotype). The level in young (3-month-old) wild-type mice is also shown as a reference ( n =3). ( c ) Cumulative number of pups are greater in transgenic animals compared with wild-type through 12 months of age ( n =4 per genotype). ( d ) Appearance of aged wild-type and transgenic ovaries (12 months). The middle section of each ovary was photographed for an unbiased comparison. Transgenic ovaries retain a larger pool of follicles appearing more active in folliculogenesis with antral follicles (arrowheads) that are more abundant in the transgenic ovaries, whereas wild-type ovaries are filled with corpora lutea. ( e ) Expression of the FOXO3 transgene by real-time PCR using construct-specific primers in wild-type (grey, no signal as expected) and transgenic (black) ovaries ( n =4 per genotype) at 9 and 12 months of age. ( f ) Expression of total Foxo3 by real-time PCR using primers common for both the transgene and the endogenous Foxo3, showing increased cumulative expression in transgenic ovaries ( n =4 per genotype). Data of panels ( a – c ; e – f ) are represented as mean values±s.e.m. * P <0.05; ** P <0.001; NS=not significant ( P >0.05). A stratified t -test was used for panels a and b ; a linear mixed-effect model was used for panel c ; and unpaired t -test was used for panels e and f . AM, morning; D, dioestrus; E, oestrus; M, metestrus; P, proestrus; PM, evening; TG, transgenic; WT, wild-type; 3M, 3 months; 9M, 9 months; 12M, 12 months. For panel d , bar, 0.2 mm. Full size image To test for a possible augmentation of fertility in aging transgenic females, we performed a long-term breeding study. Six-month-old wild-type and transgenic animals showed similar fertility, but the cumulative number of progeny from continuous breeding increased significantly in transgenic compared with wild-type females up to at least 12 months of age ( Figs. 2c , P <0.05). At 12 months, there was also an indication of greater remaining fertility in the transgenic animals (more new pups). At all stages, pups born from transgenic and wild-type females were apparently healthy and fertile ( Supplementary Fig. S1 ). In vitro fertilization studies confirmed that follicles from transgenic females were functional and could ovulate to provide normal levels of eggs competent for fertilization and blastocyst formation ( Supplementary Table S1 and Supplementary Fig. S2 ). Histological staining was consistent with gonadotropin measurements and fertility: transgenic ovaries from 12-month mice, which are usually thought of as menopausal, displayed a more dynamic activity, with greater numbers of follicles of all stages compared with wild-type ( Fig. 2d ). Consistent with an active role of the transgene in helping to maintain function in the aging ovary, real-time PCR confirmed the expression of the FOXO3 construct in 9- and 12-month-old animals ( Fig. 2e ). Once again, when using primers that could detect the mRNA from both the endogenous Foxo3 and the transgene, the overall level of expression was higher in transgenic ovaries ( Fig. 2f ). These data indicate that forced expression of active FOXO3 helps to preserve follicles, an inference that was reinforced by direct follicle counts. Follicles were divided into primordial (resting) and growing stages ( Fig. 3a ). Follicle recruitment began sharply. Two days after birth (P2), the follicles in the wild-type ovary were virtually all at the primordial stage, whereas a day later (P3) they began to be recruited to growth. Transgenic and wild-type ovaries showed the same number of primordial and growing follicles at P2 ( Fig. 3a , respectively). By P3, however, transgenic ovaries showed a trend towards slower follicle development ( Supplementary Fig. S3 shows characteristic stained sections illustrating the change from P2 to P3). Significantly more primordial follicles were present in transgenics at all ages after P2 ( P <0.001 for the overall trend, stratified t -test, Fig. 3a ). In addition, the degree of follicle activity, as measured by the number of growing follicles, was shifted to older ages in transgenics (peaking at around 6 instead of 3 months, P <0.01, stratified t -test; Fig. 3b ). 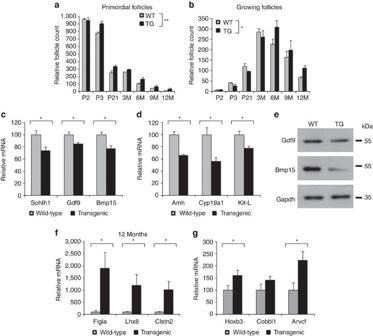Figure 3: Follicle maturation inFOXO3-transgenic mice. (a) Primordial and (b) growing follicle numbers at P2, 3 and 21, and 3, 6, 9 and 12 months, in wild-type (grey) and transgenic (black) ovaries (n=3 per genotype). With age and the approach to the mouse equivalent of menopause, follicle counts showed a larger primordial and growing follicle pool in transgenic ovaries than in wild-type. (c) Expression of oocyte and (d) somatic maturation markers at P7 (n=3 per genotype). Maturation markers are downregulated in transgenic ovaries at P7, when follicle recruitment has begun. (e) Protein level of two such markers, GDF9 and BMP15, by western blot analysis on P7 ovaries. The level of expression of these maturation markers is lower in transgenic ovaries, consistently with real-time PCR results. Expression level of Gapdh serves as a protein loading control. (f) Expression of genes associated with primordial follicles based on previous studies in 12-month-old ovaries (n=8 per genotype). Transgenic ovaries show higher levels of expression. (g) Expression of novel markers associated with a younger gene expression profile in ovaries at P7 (n=8 per genotype). Transgenic ovaries show an upregulation of these genes. P2, 2 dpn; P3, 3 dpn; P21, 21 dpn; TG, transgenic; WT, wild-type; 3M, 3 months; 6M, 6 months; 9 M, 9 months; 12M, 12 months. Data in panels (a–d,fandg) are represented as mean values±s.e.m. *P<0.05; **P<0.001. A stratifiedt-test was used for panelsaandb; unpairedt-test was used for panelsc–dandf–g. Figure 3: Follicle maturation in FOXO3 -transgenic mice. ( a ) Primordial and ( b ) growing follicle numbers at P2, 3 and 21, and 3, 6, 9 and 12 months, in wild-type (grey) and transgenic (black) ovaries ( n =3 per genotype). With age and the approach to the mouse equivalent of menopause, follicle counts showed a larger primordial and growing follicle pool in transgenic ovaries than in wild-type. ( c ) Expression of oocyte and ( d ) somatic maturation markers at P7 ( n =3 per genotype). Maturation markers are downregulated in transgenic ovaries at P7, when follicle recruitment has begun. ( e ) Protein level of two such markers, GDF9 and BMP15, by western blot analysis on P7 ovaries. The level of expression of these maturation markers is lower in transgenic ovaries, consistently with real-time PCR results. Expression level of Gapdh serves as a protein loading control. ( f ) Expression of genes associated with primordial follicles based on previous studies in 12-month-old ovaries ( n =8 per genotype). Transgenic ovaries show higher levels of expression. ( g ) Expression of novel markers associated with a younger gene expression profile in ovaries at P7 ( n =8 per genotype). Transgenic ovaries show an upregulation of these genes. P2, 2 dpn; P3, 3 dpn; P21, 21 dpn; TG, transgenic; WT, wild-type; 3M, 3 months; 6M, 6 months; 9 M, 9 months; 12M, 12 months. Data in panels ( a – d , f and g ) are represented as mean values±s.e.m. * P <0.05; ** P <0.001. A stratified t -test was used for panels a and b ; unpaired t -test was used for panels c – d and f – g . Full size image In detail, primordial follicle numbers showed a continuous trend to higher levels in transgenic mice, with fewer follicles in more advanced stages. The transgene effect remained appreciable in older ovaries (3, 6, 9 and 12 months). By 3 months, transgenic ovaries had significantly more primordial follicles ( Fig. 3a ). By 6 months, a trend was even clearer, with transgenic ovaries showing more follicles still in primordial, and by that time, more were seen in mature stages as well, and despite an increase in variance, the trend continued in 9-month-old animals ( Fig. 3a ). Twelve-month ovaries ( Fig. 3b ) showed the greatest differences. In wild-type mice only 79.6±4.5 (8%) of the initial total follicle pool remained, and those were mostly still in primary form. By contrast, transgenic ovaries showed 15% of the initial follicle pool still growing (146±22.5 remaining follicles). FOXO3 transgene preserves younger gene expression profiles To assess rate and extent of development in transgenic ovaries compared with wild-type, the expression of several oocyte and somatic genes involved in follicle maturation was evaluated. At P7, some follicles were already in the growing pool. Consistent with less follicle maturation in prepubertal transgenic mice ( Fig. 3b ), their ovaries showed significant downregulation of genes involved in follicle recruitment and/or growth, including Gdf9 , Bmp15 , Amh , Cyp19a1 (aromatase) and Kit-L [12] , [13] , [14] , [15] , [16] ( Fig. 3c ). By western blot analysis, the critical factors GDF9 and BMP15, expressed in the oocyte of growing follicles, showed protein levels consistent with gene expression ( Fig. 3e ). Band intensities showed downregulation of GDF9 and BMP15 of 32% and 74%, respectively, in transgenic compared with wild-type ovaries. Conversely, the FOXO3 transgene upregulated genes that have well-known or putative roles in early folliculogenesis, and are enriched in oocytes and/or somatic cells of primordial follicles, including Figla, Lhx8 and Clstn2 (refs 1 , 17 , 18 ) ( Fig. 3f ). In addition, expression data of transgenic and Foxo3−/− ovaries indicated that Foxo3 may partly repress Sohlh1 , a gene required for the primordial-to-primary follicle transition [17] , thus possibly affecting early follicle dynamics in a complementary fashion to Foxo3 ( Fig. 3c ; [19] , and data not shown). In addition to the increased expression of well-known primordial follicle-specific genes such as Figla and Lhx8 ( Fig. 3f ), a strong indication of a younger phenotype was also provided by the expression pattern of novel candidate youth factors that we identified by a cross-platform microarray analysis (see below). Real-time PCR validation data are shown for three of these genes, that is, the homeobox-containing gene, Hoxb3 , and the oocyte genes Cobll1 and Arvcf . Once again, these ‘youth’ genes were upregulated in transgenic ovaries, thus consistent with the transgene inducing a lower degree of follicle maturation ( Fig. 3g ). To test for direct action of the transgenic transcription factor on gene cohorts and follicle activation without the complication of accompanying wild-type alleles, we bred the transgene into a Foxo3−/− background (TG- Foxo3−/− ). Microarray analyses showed that at P14, gene lists enriched in TG- Foxo3−/− animals are indeed similar to heterozygous Foxo3+/− ovaries ( Fig. 4a , top. P <0.001), and different from Foxo3−/− ovaries ( Fig. 4a , bottom. P <0.001 in both panels). The FOXO3 transgene and the endogenous allele thus act comparably. 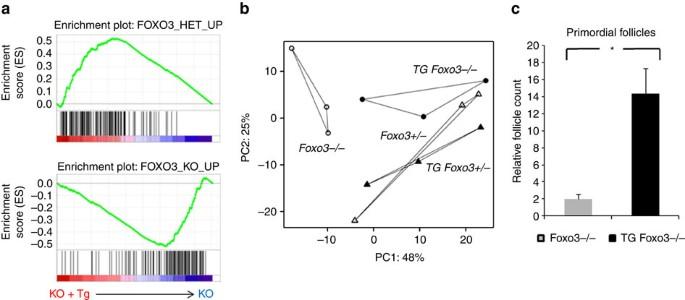Figure 4: Microarray analysis and primordial follicle count inFOXO3-transgenic ovaries. (a) Gene set enrichment analysis (GSEA) testing whether the presence of theFoxo3transgene in knockout mice induces transcriptome profiles similar to that of a single normal endogenousFoxo3allele. The horizontal axes present a ranked list of genes differentially expressed betweenFoxo3−/−ovaries carrying theFOXO3transgene compared with those not carrying it (left/red versus right/blue) (n=3 per genotype). The top list of genes enriched inFoxo3+/−heterozygous ovaries (vertical black bars of top panel) preferentially map towards the ‘red’ (transgene) side, whereas the top list of genes enriched inFoxo3−/−knockout ovaries map to the ‘blue’ (non-transgenic) side (vertical black bars of bottom panel). (b) PCA on the entire 45 k probe data set shows that TG-Foxo3−/−ovaries (black circles) are more similar toFoxo3+/−ovaries (with or without the transgene, white or black triangles, respectively) than toFoxo3−/−ovaries (white circles) (n=3 per genotype). Replicates for each condition are connected by lines. (c) Follicle count inFoxo3−/−compared with TG-Foxo3 −/−ovaries at P14 shows the presence of some primordial follicles in transgenic ovaries, while no primordial follicles could be found in knockout ovaries (n=3 per genotype). Data are represented as mean values±s.e.m. *P<0.05, unpairedt-test. Figure 4: Microarray analysis and primordial follicle count in FOXO3 -transgenic ovaries. ( a ) Gene set enrichment analysis (GSEA) testing whether the presence of the Foxo3 transgene in knockout mice induces transcriptome profiles similar to that of a single normal endogenous Foxo3 allele. The horizontal axes present a ranked list of genes differentially expressed between Foxo3−/− ovaries carrying the FOXO3 transgene compared with those not carrying it (left/red versus right/blue) ( n =3 per genotype). The top list of genes enriched in Foxo3+/− heterozygous ovaries (vertical black bars of top panel) preferentially map towards the ‘red’ (transgene) side, whereas the top list of genes enriched in Foxo3−/− knockout ovaries map to the ‘blue’ (non-transgenic) side (vertical black bars of bottom panel). ( b ) PCA on the entire 45 k probe data set shows that TG- Foxo3−/− ovaries (black circles) are more similar to Foxo3+/− ovaries (with or without the transgene, white or black triangles, respectively) than to Foxo3−/− ovaries (white circles) ( n =3 per genotype). Replicates for each condition are connected by lines. ( c ) Follicle count in Foxo3−/− compared with TG- Foxo3 −/− ovaries at P14 shows the presence of some primordial follicles in transgenic ovaries, while no primordial follicles could be found in knockout ovaries ( n =3 per genotype). Data are represented as mean values±s.e.m. * P <0.05, unpaired t -test. Full size image Principal component analysis (PCA) gave consistent results ( Fig. 4b ). Along the first principal component (48% of global transcriptional variance) TG- Foxo3−/− (black symbols) and TG- Foxo3+/− ovaries (black triangles) colocalized with the non-transgenic Foxo3+/− (white triangles) and separated from Foxo3−/− ovaries (white circles). Along the second principal component (25% of variance), however, TG- Foxo3−/− ovaries were clustered with Foxo3−/− . Thus, much though not all gene expression was rescued by the transgene. To test the effect of the FOXO3 transgene on ovarian maturation, expression results were also mapped onto a PCA space constructed from 521 ‘developmental’ genes that showed the greatest variation across 141 gonadal samples in previous studies [18] . We had shown that PCA on these gonadal samples can discriminate the course of development and aging. Foxo3−/− ovaries were located nearer ‘older’ ovaries (right side) than were Foxo3 +/− ovaries, and Foxo3−/− ovaries carrying the transgene were clearly located closer to the ‘younger’ (left) cluster ( Supplementary Fig. S4a,b ). Consistent with microarray data, targeted counting found that by P14 Foxo3−/− animals, in agreement with the report by Castrillon et al. [6] , had virtually no remaining primordial follicles (0.002%), whereas the TG- Foxo3−/− ovaries still retained a proportion of the original primordial follicles pool (1.5%) ( Fig. 4c and Supplementary Fig. S5 ). Transgenic ovary profiles were also enriched for specific genes that we found specifically more expressed either in younger or in older ovaries ( Supplementary Fig. S6a ). ‘Youthful’ genes included Hoxa9 , Hoxb3 , Cobll1 , Pcdh10 and Arvcf (cf. Fig. 3g ); ‘aging’ genes included Adcy7 , Cidea , Bdnf and Foxc2 . These findings can be correlated with the dynamics of follicle fate. In mice as in humans, the follicle pool formed around birth in females represents an essentially non-renewing population [3] , [4] . It has been proposed that some follicular renewal occurs in adult mice [20] , [21] ; but even including such a contribution, follicle numbers progressively decline, leading to menopause [22] . In this study, follicle numbers confirmed a continuously larger reserve of primordial follicles in the transgenic ovaries. Furthermore, 9-month-old transgenic animals showed lower age-related increases in the levels of gonadotropins, and substantially higher numbers of preantral and antral stage follicles. We infer that active FOXO3 helps to preserve oocytes in a competent state, and can rationalize the striking increase in fertility of transgenic females starting from 7 months of age, yielding 31–49% more viable embryos at every time point, even at 12 months. There is a hint that the transgenic females may also have extended reproductive lifespan compared with wild-type (note the differential slope between 11 and 12 months in Fig. 2c ). However, more extensive studies would be required to test that possibility further, and they are made difficult by the less robust mating observed with all female mice by that age. One would expect that Foxo3 would have its effects through an action at transcription, and indeed the transgene induces a younger gene expression profile ( Supplementary Fig. S4 ). Both timing and level of Foxo3 expression are likely to be important, also indicated by findings that a construct similar to the one described here but expressed from a Zp3 promoter resulted in severely delayed follicular development and infertility [23] . As Zp3 is preferentially active in growing oocytes [24] , the Zp3-Foxo3 transgene presumably misexpresses FOXO3 at a stage of ongoing oocyte growth, which may disrupt folliculogenesis. In sharp contrast, Kit -like Foxo3 is selectively expressed in oocytes of primordial and primary follicles [25] (cf. GEO data set GSE3351). Accordingly, the Kit promoter included in our transgene has greatest expression in the newborn ovary [10] and thus reproduces the natural Foxo3 expression pattern, whereas the engineered protein is expected to increase FOXO3 action in blocking oocyte growth before it starts. This block is possibly relieved, in part, by downregulation of the transgene-associated Kit promoter via factors that reproduce endogenous Kit downregulation in early growing follicles. In addition, although transgene expression is targeted appropriately to the oocyte of primordial follicles by the use of the Kit promoter [10] , the exact timing of expression may vary somewhat from that of the endogenous Foxo3 promoter and may reduce the effectiveness of the Foxo3 transgene. As an additional possible weakness of our Foxo3 -transgenic model, the alanine substitutions at phosphorylation sites of the transgenic FOXO3 protein may disturb positive functional interactions. Based on its ability to help conserve an active, more ‘youthful’ follicle reserve, active Foxo3 promotes long-term maintenance of the follicle pool. Ovarian follicle dynamics may thus follow relatively simple genetic mechanisms in mammals. It may be relevant that comparable effects on follicle levels were previously obtained by ablating the pro-apoptotic Bax [26] , [27] . The relatively specific and positive effects of Foxo3 on follicles make it an especially intriguing point for possible agonist intervention to alleviate physiological decline of female fertility. Mouse strains and husbandry The transgene was generated by inserting a mutagenized human FOXO3 sequence between a 6.3-kb mouse Kit promoter and a 0.6-kb 3′-flanking region from the human growth hormone ( GH1 ) gene in a pUC18 vector (a generous gift of Dr J. A. Flaws). This construct was previously used to drive ovarian expression of a Bcl2 transgene with minimal or no overexpression in other tissues [26] . Mutagenesis of the human FOXO3 sequence involved the conversion of the codons for threonine 32 and serines 253, 315, 318, 321 and 325 into alanine by stepwise standard PCR-mediated replacement and sequence verification. Transient transfection assays in several cell lines showed predominantly nuclear staining for the mutagenized FOXO3 protein (not shown). The construct spanning 12 kb was injected into pronuclei of FVB/N mice (Transgenic Mouse Core, Baylor College of Medicine). We obtained Foxo3−/− mice from the Mutant Mouse Regional Resource Center (UC Davis, CA, USA). All mouse strains were maintained on a FVB/N genetic background. Mice were euthanized ethically according to ACUC-approved NIA Standard Operation Procedures. Gonads were collected at 0, 2, 3, 7, 14 and 21 days, and 3, 6, 9 and 12 months. The study of the oestrous period was performed on five females for each genotype. Females at 3 (used as reference) and 9 months of age were monitored for the entire oestrous period, which lasted 5 days. Females were exposed to mouse pheromones (male bedding) to promote cycling. Every morning vaginal swabs were performed and vaginal smears were analysed by hematoxylin and eosin staining. For the entire period, blood was collected from each female twice a day (mornings and evenings) according to ACUC-approved NIA Standard Operation Procedures. Gonadotropin measurements Gonadotropins were measured on coded samples using specific RIAs by Ligand Assay and Analysis Core of the University of Virginia Center for Research in Reproduction. Transgenic and control females ( n =4 per genotype) were housed together with wild-type males from the age of 5 months onwards, and their fertility (date of delivery and number of pups) recorded until they were 12 months old. All procedures and protocols were conducted in accordance with the guidelines approved by the Animal Care and Use Committee of the NIA Intramural Research Program (ASP 283-LG-2013). In vitro fertilization Young female mice were superovulated by intraperitoneal administrations of 5 IU pregnant mare’s serum on day 1 and 5 IU human chorionic gonadotropin 46–48 h later. Fifteen to 17 h following human chorionic gonadotropin injection, mice were euthanized by cervical dislocation and the oviducts dissected out. Cumulus–oocyte complexes were collected from oviducts and cultured in IVF medium in 5% CO 2 at 37 C°. Unfertilized eggs were released into cell culture media and collected. Male mice that had not been mated for more than 2 weeks were euthanized and sperm collected from the epididymis. The sperm was incubated for 20–30 min in capacitation medium in 5% CO 2 at 37 C°. Capacitated spermatozoa (concentration 1–2 × 1,000,000) were inseminated into cumulus–oocyte complexes drops. After incubation for 5–6 h, the oocytes were washed through several changes of Hepes-medium followed by at least one wash in culture medium. Embryos were then maintained in vitro in microdrops (25 ml) of KSOM culture medium for up to 96 h. Every 24 h, dishes were rapidly examined for embryonic development. RNA expression analysis Real-time PCR assays (TaqMan, Applied Biosystems) was performed on three biological replicates per genotype. For each replicate, five ovaries were pooled and total RNA extracted (Total RNA Extraction kit, RBC). RNA was then amplified using a Pico Ovation kit (NuGEN) followed by affinity purification (Zymo Research). Quantitative real-time PCR was performed using an ABI 7900HT system (Applied Biosystems). Normalization was done by scaling to expression of Sdha using the following TaqMan probes: Amh (Mm00431795_g1); Arvcf (Mm01344997_g1); Bmp15 (Mm00437797_m1); Clstn2 (Mm00502574_m1); Cobll1 (forward primer: 5′-GGTAATTTT CCATCAATCAACCTTTG-3′; reverse primer: 5′-CCGCAATGCAACCAACAAT-3′; FAM probe: 5′-ATGTCCCAGCCCAGC-3′), Cyp19a1 (Mm00484049_m1); Figla (Mm00488823_m1); Foxo3 (Mm01185722_m1); transgenic FOXO3 (forward primer: 5′-CCGGCTGGAAGAACTCCAT-3′; reverse primer: 5′-CCGCATGAATCGACTATGCA-3′; FAM probe: 5′-CGGCACAACCTGTCA-3′); Gdf9 (Mm00433565_m1); Hoxb3 (forward primer: 5′-TCTTGTTGCACTTGGAGTTTACATT-3′; reverse primer: 5′-TGAGCGAAGCTGGACTTTCTG-3′; FAM probe: 5′-CAACTGTGAGAGATGTCT-3′); Kitl (Mm00442972_m1); Lhx8 (Mm00802919_m1); Sdha (Mm01352366_m1); Sohlh1 (Mm01338424_g1). Microarray analysis For each genotype, gonads from each of three pups were separately processed to provide replicates. Total RNA was extracted, amplified, purified (as above) and labelled for MouseWG-6 v2 Expression BeadChip arrays (Illumina). In order to test if the global transcriptional profile of Foxo3−/− mice carrying the transgene had become similar to the normal profile compared with Foxo3−/− mice without the transgene, we carried out unsupervised PCA on all 45 k probe levels normalized by Illumina proprietary software. In particular, we used the svd function in R to map the transgenic ovaries onto PCA space constructed based on the non-transgenic ovaries ( Fig. 3b ). This emphasized differences between Foxo3−/− and Foxo3+/− ovaries rather than between the presence or absence of the transgene. In order to test for an effect of the FOXO3 transgene on ovarian maturation, we carried out PCA on our gonadal development data set and mapped a wide range of other gonadal samples that were published by others, as previously reported [18] . All these samples ( N =141) were studied on the same Affymetrix platform. In order to map our current samples (which were done on a different platform, Illumina), we modified the procedure by adding a normalization step (centring to the median and reducing by the median absolute deviation from the median) and restricting the list of genes to the intersection between the 6 k probes that showed strongest differential expression in the Affymetrix samples and the top 5 k probes that showed strongest differential expression in the Illumina samples according to Focus total variance analysis [28] (the thresholds corresponded to similar statistical cutoffs). The shared list of 521 non-redundant genes was used to carry out PCA and ‘PCA mapping’ on the various samples (using svd in R, as above). The PCA results are shown in Supplementary Fig. S4 . The 48 genes that best discriminate our Foxo3−/− and FOXO3 -transgenic samples along PC1 (values above versus below PC1 cutoff of 0.5 in Supplementary Fig. S4b ) were obtained using predictive analysis of microarrays [29] ( Supplementary Fig. S6 ). Our microarray data set can be downloaded from the public website, http://www.ncbi.nlm.nih.gov/geo , via accession number GSE45389 . Histological preparation and immunohistochemistry Gonads were fixed in Bouin solution for 2 h for histological evaluation and follicle count. Gonads assigned for immunohistochemistry were fixed in 4% paraformaldehyde-phosphate-buffered saline (PBS). After fixation gonads were embedded in paraffin and sectioned at 3μm, follicle counts were carried out on hematoxylin- and eosin-stained sections. Primordial follicles were defined as having an oocyte surrounded by a single layer of flat granulosa cells. All other follicles at more advanced stages of maturation were grouped and defined as growing follicles. Ovaries from three gonads for each genotype and at each stage were analysed; every tenth section was photographed and follicles were counted. For immunohistochemistry, ovary sections were deparaffinized in toluene and rehydrated using sequential washes and decreasing alcohol concentrations (100–95–70–50% ethanol–PBS). Heath-mediated antigen retrieval was performed in a EMS-820 precision-pulsed laboratory microwave oven (Electron Microscopy Sciences) by heating the slides in 10 mM citrate buffer, pH 6.0 at 90 °C for 5–10 min. Primary antibodies for Foxo3 (Abcam) andVasa (BP Pharmingen) were each diluted 1:100, and incubated overnight at 4 °C. Secondary antibodies from Alexa Fluor (Invitrogen, dilution 1:500) were incubated at room temperature for 30 min. The slides were incubated with DAPI (Dojindo Molecular Technologies, 100 ng ml −1 ) at room temperature for 15 min, and finally mounted with Prolong Gold Antifade solution (Invitrogen). Images were taken with a Deltavision fluorescence microscope (Applied Precision) and processed using Adobe Photoshop CS. Western blotting Ovaries were homogenized (Precellys 24, Bertin, France) and protein extracted in Radio Immuno Precipitation Assay buffer supplemented with phosphatase inhibitors (Roche Diagnostic). The protein content was determined using the Bradford assay on a Victor 3 V Reader (PerkinElmer). Equal amounts of protein (10 μg) was fractionated in 8–16% SDS–polyacrylamide gel electrophoresis and analysed by western blotting with the following antibodies: Foxo3 (Cell Signaling, dil 1:1,000), Amh (Santa Cruz, dil 1:500), Bmp15 (Abcam, dil 1:500), Gdf9 (Abcam, dil 1:500), β-actin (Bethyl, dil 1:2,000) and Gapdh (Santa Cruz, dil 1:1,000). Band intensity analyses were performed using Molecular Imaging Software (ver. 4.0.5; Kodak). Statistical analyses For comparison of gonadotropin levels and follicle counts, statistical significance was calculated using the SAS program. Significance of cumulative number of progeny was calculated using a linear mixed-effect model (implemented in SAS). For gene expression using real-time PCR, statistical analysis was performed by the unpaired t -test (GraphPad). Accession codes: The microarray data have been deposited in Gene Expression Omnibus (GEO) under the accession code GSE45389 . How to cite this article: Pelosi, E. et al. Constitutively active Foxo3 in oocytes preserves ovarian reserve in mice. Nat. Commun. 4:1843 doi: 10.1038/ncomms2861 (2013).